Vaginal type-II mucosa is an inductive site for primary CD8+T-cell mucosal immunity The structured lymphoid tissues are considered the only inductive sites where primary T-cell immune responses occur. The naïve T cells in structured lymphoid tissues, once being primed by antigen-bearing dendritic cells, differentiate into memory T cells and traffic back to the mucosal sites through the bloodstream. Contrary to this belief, here we show that the vaginal type-II mucosa itself, despite the lack of structured lymphoid tissues, can act as an inductive site during primary CD8 + T-cell immune responses. We provide evidence that the vaginal mucosa supports both the local immune priming of naïve CD8 + T cells and the local expansion of antigen-specific CD8 + T cells, thereby demonstrating a different paradigm for primary mucosal T-cell immune induction. Lying at the interface between host and environment, the mucosal tissue acts as the port of entry for multiple pathogens. During viral transmission through mucosal tissues, the presence of local antigen (Ag)-specific immune cells is considered to help control infections by multiple viruses, such as influenza virus (Flu) [1] , [2] , [3] , human immunodeficiency virus (HIV) [4] , [5] , [6] , [7] , [8] , Simian immunodeficiency virus (SIV) [9] , [10] , [11] and herpes simplex virus (HSV) [12] , [13] , [14] , [15] . Although the mucosal local Ag-specific T cells play an important role to protect against viral transmission, the mechanisms through which the local Ag-specific T-cell immunity can be generated in mucosal tissues, especially in type-II mucosa (found in vagina, glans penis and oesophagus) [16] , [17] , [18] , [19] , remain to be elucidated. It is widely believed that primary immune T-cell induction in type-II mucosa occurs only in the draining lymph nodes (DLNs) but not in the mucosa itself due to a lack of mucosa-associated lymphoid tissue (MALT) or secondary lymphoid tissues [16] , [17] , [18] , [19] . In this process, the naïve T cells in DLNs are primed by the Ag-bearing dendritic cells (DCs) migrating from the Ag-exposed mucosa and differentiate into memory T cells that are then able to traffic back to mucosal sites through the bloodstream [20] , [21] , [22] , [23] . It has been shown that local secondary immune responses can protect against viral infection [24] , [25] , [26] , and that protective vaginal immunity can occur in lymph node-deficient mice [13] , as well as that lymphoid clusters can form in virus-infected vaginal mucosa [15] . However, whether a primary immune response can be induced locally in the type-II mucosal tissues without help from any distant tissue or lymphoid site remains a fundamental question to be answered. In the current study, we develop a unique dual-transfer model, by which we clearly demonstrate that adoptively transferred naïve OT-I CD8 + T cells are activated in the vaginal mucosa but not in the DLNs 24 h after intravaginally (Ivag) immunization under conditions where cells from the circulation or DLNs cannot reach the vaginal mucosa. Even without adoptive transfer, Ag-specific CD8 + T-cell activation is found to occur locally in the vaginal mucosa after vaginal immunization before it occurs in DLNs. In addition, the immunized vaginal tissue can induce naïve OT-I CD8 + T-cell activation that is largely dependent on local antigen-presenting cells (APCs). Finally, vaginal mucosa also supports the local expansion of Ag-specific CD8 + T cells. In conclusion, we present an evidence of a new paradigm for primary CD8 + T-cell immune induction in type-II mucosa of the vagina, one that occurs locally without the help of draining LNs, MALT or any other tissue site of priming, thereby providing a new rationale for local mucosal immunization. DLN-independent priming of CD8 + T cells in vaginal mucosa Our study started with our observation that Ivag-immunized LN-deficient lymphotoxin-alpha-knockout (LTα KO) mice [27] , [28] could still be immunized Ivag despite lack of DLNs. To test the necessity of DLNs for vaginal CD8 + T-cell immune induction, we used a replication-deficient adenovirus-5-expressing the hen ovalbumin immunodominant K b -restricted SIINFEKL peptide (rAd5-SIINFEKL) to Ivag immunize the LN-deficient lymphotoxin-alpha-knockout (LTα KO) mice [27] , [28] ( Fig. 1a ) and measured the vaginal SIINFEKL-specific CD8 + T cells 14 days post immunization (PI). Significantly elevated levels of SIINFEKL-specific CD8 + T cells could be detected in the vaginal mucosa of LTα KO mice ( Fig. 1b,c ), although the percentage was lower than that in wild-type (WT) animals. To understand the vaginal T-cell distribution after Ivag immunization, we examined the vaginal tissue sections and found that immunization-induced CD3 + cell clusters formed in both WT and LTα KO mice ( Fig. 1d ). To further identify the phenotype of cluster-forming cells, we stained CD8 and CD11c on the consecutively cut tissue sections right next to each other. The adjacent tissue section staining showed that the CD3 + cell clusters in the immunized mice also contained CD8 + and CD11c + cells ( Fig. 1d ). In contrast to the immunized mice, the vaginal CD3 + cells in naïve animals did not form clusters, but rather they were present sporadically as isolated cells in lamina propria (LP) and epithelium ( Fig. 1d ). These results clearly demonstrated that primary Ivag immunization could induce the LN-independent Ag-specific CD8 + T-cell immune response associated with the immune cell aggregation, that is, the formation of inducible vaginal lymphoid tissue (IVALT). Although the IVALT-associated Ag-specific CD8 + T-cell response can be induced in the vaginal mucosa independent of LNs, consistent with the recent findings on protective immunity of Roth et al . [13] , we still do not know whether these Ag-specific CD8 + T cells are derived from the primed local naïve T cells in the vaginal mucosa or they migrate from other non-lymphoid tissue compartments, such as the liver [29] , [30] , [31] . To test whether or not the vaginal mucosa itself could act as an inductive site for the primary CD8 + T-cell immune responses, we wanted to determine whether a primary CD8 + T-cell response could be generated locally in the vaginal mucosa of WT mice. 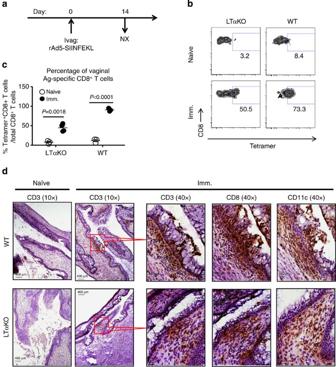Figure 1: Vaginal Ag-specific CD8+T-cell immune responses in LTα KO LN-deficient mice. (a–c) The percentage of SIINFEKL-specific CD8+T cells in the vaginal mucosa of both LTα KO, LN-deficient mice and WT mice. This is representative of two independently repeated experiments (n=3 per naïve control group;n=4 per immunized group) with the same results. (a) Experimental design. (b) The gating strategy. (c) The percentage (mean±s.e.m.) of SIINFEKL-specific vaginal CD8+T cells in each group. ThePvalue was generated using Student’st-test. (d) Representative IHC staining showing the formation of immune cell clusters containing CD3+, CD8+and CD11c+cells in the immunized WT and LTαKO mice. Scale bar: 100 μm in × 40 photomicrographs; 400 μm in × 10 photomicrographs. Imm, immunized. Figure 1: Vaginal Ag-specific CD8 + T-cell immune responses in LTα KO LN-deficient mice. ( a – c ) The percentage of SIINFEKL-specific CD8 + T cells in the vaginal mucosa of both LTα KO, LN-deficient mice and WT mice. This is representative of two independently repeated experiments ( n =3 per naïve control group; n =4 per immunized group) with the same results. ( a ) Experimental design. ( b ) The gating strategy. ( c ) The percentage (mean±s.e.m.) of SIINFEKL-specific vaginal CD8 + T cells in each group. The P value was generated using Student’s t -test. ( d ) Representative IHC staining showing the formation of immune cell clusters containing CD3 + , CD8 + and CD11c + cells in the immunized WT and LTαKO mice. Scale bar: 100 μm in × 40 photomicrographs; 400 μm in × 10 photomicrographs. Imm, immunized. Full size image The availability of naïve CD8 + T cells in vaginal mucosa Because the availability of naïve T cells is a prerequisite for the generation of primary T-cell immune responses, we first assessed whether naïve CD8 + T cells were present in the vaginal mucosa. To ensure the CD8 + T cells we identified from the digested vaginal tissue were the interstitial cells, we intravenously (i.v.) injected fluorochrome-labelled Thy1.2 antibody at a dose of 25 ng per mouse that could stain all the T cells in the blood collected from retro-orbital plexus within 1 min ( Supplementary Fig. 1a ), which means that all the vasculature T cells can be stained by this method. Using the intravascular T-cell staining [32] , we can clearly distinguish the interstitial T cells from the blood T cells, although some of the tissue-residing cells might be stained by the antibody that leaks out from the capillaries, so the unstained cells represent a lower limit on the number of tissue-residing cells. In digested vaginal tissues, we found that around 86% (median=86.7%) of naïve CD8 + T cells (CD62L high /CD44 low ) were present extravascularly, that is, in the vaginal mucosal parenchyma, but not in associated vasculature ( Supplementary Fig. 1a,b ). We then examined the phenotype of vaginal CD8 + T cells from mice treated either with or without FTY720, a sphingosine-1-phosphate receptor agonist, which inhibits lymphocyte egress from both thymus and lymph nodes [33] ( Fig. 2 ). In FTY720-untreated mice, 44% (44.7%±4.1%; mean±s.e.m.) of vaginal CD8 + T cells showed a naïve phenotype characterized as CD62L + , CD44 low and lacking CD25 and CD69 expression ( Fig. 2b,c ). Four days after FTY720 treatment, the naïve CD8 + T-cell population in the vaginal mucosa was lost ( Fig. 2b,c ). 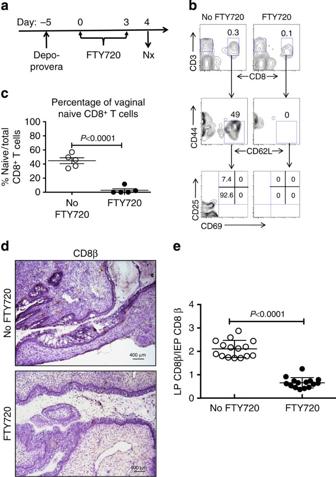Figure 2: The phenotype and distribution of CD8+T cells in vaginal mucosa of WT mice with or without FTY720 treatment. (a–c) The naïve CD8+T cells in the vaginal mucosa of WT mice with depo-provera-synchronized oestrous cycle. This is representative of three independently repeated experiments (n=5) with the same results. (a) Experimental design. (b) The gating strategy to identify vaginal naïve CD8+T cells. (c) The percentage (mean±s.e.m.) of naïve CD8+T cells in vaginal mucosa with or without FTY720 treatment. (d,e) Representative results of vaginal IHC staining showing the distribution of C8β+cells in vaginal LP and epithelium. (d) Representative IHC photomicrographs showing the CD8 β+cell in both vaginal epithelium and LP of the mice treated either with or without FTY720 (Scale bar, 400 μm). (e) The ratio of LP C8β+cells/IEP C8β+cells summarized from the pool of three independently repeated experiments (n=15). The numbers of LP and IEP C8β+cells were counted from three vaginal tissue sections from each animal. To avoid counting the same cell multiple times on adjacent tissue sections, we selected the slides with the vaginal tissue sections that were cut 25 μm apart based on the diameter of T cells (5–20 μm) (ref.63). ThePvalue was generated using a Student’st-test. Figure 2: The phenotype and distribution of CD8 + T cells in vaginal mucosa of WT mice with or without FTY720 treatment. ( a – c ) The naïve CD8 + T cells in the vaginal mucosa of WT mice with depo-provera-synchronized oestrous cycle. This is representative of three independently repeated experiments ( n =5) with the same results. ( a ) Experimental design. ( b ) The gating strategy to identify vaginal naïve CD8 + T cells. ( c ) The percentage (mean±s.e.m.) of naïve CD8 + T cells in vaginal mucosa with or without FTY720 treatment. ( d , e ) Representative results of vaginal IHC staining showing the distribution of C8β + cells in vaginal LP and epithelium. ( d ) Representative IHC photomicrographs showing the CD8 β + cell in both vaginal epithelium and LP of the mice treated either with or without FTY720 (Scale bar, 400 μm). ( e ) The ratio of LP C8β + cells/IEP C8β + cells summarized from the pool of three independently repeated experiments ( n =15). The numbers of LP and IEP C8β + cells were counted from three vaginal tissue sections from each animal. To avoid counting the same cell multiple times on adjacent tissue sections, we selected the slides with the vaginal tissue sections that were cut 25 μm apart based on the diameter of T cells (5–20 μm) (ref. 63 ). The P value was generated using a Student’s t -test. Full size image To determine the location of CD8 + T cells in vaginal mucosa, we assayed the number of vaginal CD8β + cells in the mice either with or without FTY720 treatment by immunohistochemistry (IHC; Fig. 2d,e ). In FTY720-treated animals, the ratio of LP CD8β + cells/intraepithelial (IEP) CD8β + cells significantly decreased ( P <0.0001 by a Student’s t -test) from 2.03±0.097 (mean±s.e.m.) to 0.53±0.059 ( Fig. 2d,e ). Although it is difficult to count and compare the absolute number of total CD8 + T cell in both LP and IEP due to the sporadic cell distribution, the lower LP/IEP ratio in FTY720-treated animals is highly suggestive of FTY720-induced vaginal naïve T-cell depletion occurring to a greater extent in the LP. Even though naïve lymphocytes are known to preferentially recirculate among the secondary lymphoid organs [34] , [35] , there is an increasing evidence showing that CD8 + recent thymic emigrants migrate directly into the small intestine and that naïve T and B lymphocytes are present in multiple peripheral tissue compartments [36] , [37] , [38] , [39] . Therefore, our data demonstrated that naïve CD8 + T cells routinely migrated into the vaginal mucosal LP and the maintenance of this population depended on the lymphocyte recirculation or replenishment from the bloodstream. Naïve T-cell vaginal mucosal priming 24 h post Ivag vaccine To determine whether the naïve CD8 + T cells could be primed locally in the vaginal mucosa of WT mice, independent of DLNs, we developed a dual-transfer model ( Fig. 3a ). We isolated CD8 + T cells from Rag1 KO, OT-I transgenic C57BL/6 mice that solely express a T-cell receptor (TCR) recognizing the ovalbumin peptide SIINFEKL-H-2K b complex. We depleted CD44 high cells from the OT-I CD8 + T cells to enrich the naïve population (CD44 low and CD62L + ) to 98.5% ( Fig. 3a ). Identical aliquots of the naïve OT-I CD8 + T cells were labelled with either carboxyfluorescein succinimidyl ester (CFSE; green) or violet dye and adoptively transferred either Ivag or i.v., respectively, into the same recipient mouse that had been Ivag immunized either 8 h ( Fig. 3b ) or 32 h ( Fig. 4a ) earlier with SIINFEKL peptide plus DOTAP, a cationic liposome facilitating major histocompatibility complex-I-restricted Ag presentation, and mutant labile toxin (mLT), a mucosal adjuvant. To further block lymphocyte recirculation, we also gave each mouse FTY720 at 24 h before euthanasia, which decreased the number of blood CD8 + T cells to background levels from 8–24 h post treatment ( Fig. 3a ). 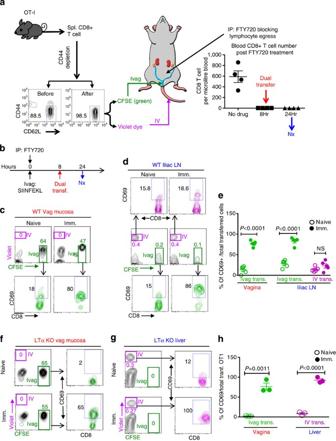Figure 3: The CD69 expression of Ivag- versus i.v.-transferred naïve OT-I CD8+T cells in WT and LN-deficient LTαKO mice at 24 h PI. (a) The dual-transfer model. (b)The experimental design. (c–e) The CD69 expression of transferred naïve OT-I CD8+T cells in the vaginal mucosa and iliac LNs of WT mice. This is representative of three independently repeated experiments (n=5 for WT animals;n=3 for LTαKO animals) with the same results. (c) The total and CD69-expressing transferred naïve OT-I CD8+T cell in the vaginal mucosa. (d) The total and CD69-expressing transferred naïve OT-I CD8+T cell in the iliac LNs. (e) The percentage (mean±s.e.m.) of CD69 expression in each group. (f–h) The total and CD69-expressing transferred naïve OT-I CD8+T cells in the vaginal mucosa and the liver of LN-deficient LTαKO mice. This is representative of two independently repeated experiments with the same results. (f) The total and CD69-expressing transferred naïve OT-I CD8+T cell in vaginal mucosa of LTα KO mice. (g) The total and CD69-expressing transferred naïve OT-I CD8+T cell in liver of LTαKO mice. (h) The percentage (mean±s.e.m.) of CD69 expression in each group. ThePvalue was generated using a Student’st-test. Imm., immunized. Figure 3: The CD69 expression of Ivag- versus i.v.-transferred naïve OT-I CD8 + T cells in WT and LN-deficient LTαKO mice at 24 h PI. ( a ) The dual-transfer model. ( b )The experimental design. ( c – e ) The CD69 expression of transferred naïve OT-I CD8 + T cells in the vaginal mucosa and iliac LNs of WT mice. This is representative of three independently repeated experiments ( n =5 for WT animals; n =3 for LTαKO animals) with the same results. ( c ) The total and CD69-expressing transferred naïve OT-I CD8 + T cell in the vaginal mucosa. ( d ) The total and CD69-expressing transferred naïve OT-I CD8 + T cell in the iliac LNs. ( e ) The percentage (mean±s.e.m.) of CD69 expression in each group. ( f – h ) The total and CD69-expressing transferred naïve OT-I CD8 + T cells in the vaginal mucosa and the liver of LN-deficient LTαKO mice. This is representative of two independently repeated experiments with the same results. ( f ) The total and CD69-expressing transferred naïve OT-I CD8 + T cell in vaginal mucosa of LTα KO mice. ( g ) The total and CD69-expressing transferred naïve OT-I CD8 + T cell in liver of LTαKO mice. ( h ) The percentage (mean±s.e.m.) of CD69 expression in each group. The P value was generated using a Student’s t -test. Imm., immunized. 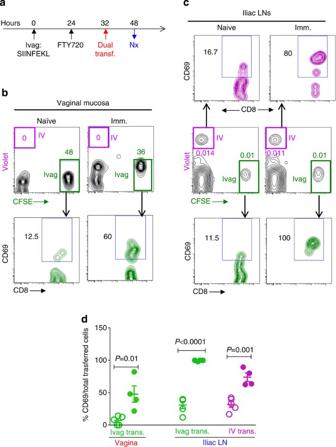Figure 4: The CD69 expression of Ivag- versus i.v.-transferred OT-I CD8+T cells in vaginal mucosa and iliac LNs at 48 h PI. (a) The experimental design. (b) The total and CD69-expressing transferred OT-I CD8+T cells in vaginal mucosa. (c) The total and CD69-expressing transferred OT-I CD8+T cells in iliac LNs. (d) The percentage (mean±s.e.m.) of CD69+OT-I CD8+T cells in each group. This is representative of two independently repeated experiments (n=5 per naïve group;n=4 per immunized group) with the same results.Pvalue was generated using a Student’st-test. Imm., immunized. Full size image Figure 4: The CD69 expression of Ivag- versus i.v.-transferred OT-I CD8 + T cells in vaginal mucosa and iliac LNs at 48 h PI. ( a ) The experimental design. ( b ) The total and CD69-expressing transferred OT-I CD8 + T cells in vaginal mucosa. ( c ) The total and CD69-expressing transferred OT-I CD8 + T cells in iliac LNs. ( d ) The percentage (mean±s.e.m.) of CD69 + OT-I CD8 + T cells in each group. This is representative of two independently repeated experiments ( n =5 per naïve group; n =4 per immunized group) with the same results. P value was generated using a Student’s t -test. Imm., immunized. Full size image To validate the reliability of our dual-transfer system, we tested the effectiveness of T-cell recirculation blockage mediated by FTY720 treatment. WT mice received FTY720 IP injection followed by i.v.-transferred, CFSE-labelled naïve CD8 + T cells (5 × 10 6 per mouse) at 8 h after FTY720 treatment. Sixteen hours after adoptive transfer, we collected and combined five vaginal tissues from the mice that had received either naïve CD8 + T cells or naïve CD8 + T cells plus FTY720 or PBS. The transferred naïve CD8 + T cells were examined using flow cytometry and no CFSE + events were noted in the vaginal tissues from the FTY720-treated mice, whereas they were clearly detected in the absence of FTY720. This is direct evidence that FTY720 completely blocked the naïve CD8 + T-cell vaginal infiltration from the blood stream ( Supplementary Fig. 2 ). We investigated the vaginal CD8 + T-cell immune priming at 24 h PI (16 h after dual transfer; Fig. 3b ). In the vaginal mucosa, the only detectable transferred population was the green CFSE-labelled cell population injected directly into the vaginal mucosa ( Fig. 3c ). The percentage of green CFSE-labelled OT-I CD8 + T cells out of total vaginal CD8 + T cells was about 50% (51.2%±4.9%; mean±s.e.m. ), which means the number of transferred naïve CD8 + T cells within the vaginal tissue was similar to that of the endogenous CD8 + T cells (that is, physiological levels; Fig. 3c ). The CD69 expression of Ivag-transferred cells was significantly higher in the Ivag-immunized mice (84%±2.9%; mean±s.e.m.) than the naïve control animals (10.9%±2.7%; mean±s.e.m. ; P <0.0001 by a Student’s t -test; Fig. 3c,e ), indicating that these cells were primed by the Ivag immunization. Since the violet-labelled i.v.-transferred cells were not detectable in the vaginal mucosa 24 h after immunization ( Fig. 3c ), there were no transferred T cells entering the vaginal mucosa through the bloodstream in the presence of FTY720. Therefore, the green CD69 + Ivag-transferred cells would not yet have been able to traffic back to vaginal mucosa from the DLNs (or any other tissue) where they could potentially have been activated. Thus, the CD69 + green Ivag-transferred cells in the vaginal mucosa had to be primed locally. For comparison, the draining iliac LN contained both i.v.-transferred and Ivag-transferred cells ( Fig. 3d ). The i.v.-transferred cells showed similar low levels of CD69 expression in the immunized as in the naïve animals, indicating a lack of priming in the DLN by the Ivag immunization at 24 h. In contrast, the CD69 expression of the green Ivag-transferred cells was significantly higher in the immunized mice than unimmunized mice. Since the violet-labelled i.v.-transferred cells had not been activated in the iliac LN by 24 h PI, those green CD69 + Ivag-transferred cells in iliac LNs would not have been activated in the LNs, but should be the ones activated in the vaginal mucosa that then migrated into the DLNs. For further confirmation, we also performed a similar dual-transfer study in LN-deficient lymphotoxin-alpha-knockout (LTα KO) mice [27] , [28] ( Fig. 3f–h ). Similar to what was observed in WT mice, the green Ivag-transferred cells within the vaginal mucosa were activated at 24 h PI without any evidence of any T-cell vaginal homing through the bloodstream (violet i.v.-transferred cells; Fig. 3f,h ). Because the LTα KO mice don’t develop any LNs, we checked the liver that also possesses multiple immune functions [29] . Similar to what has been shown by other groups [30] , [31] , the immune priming, characterized by the expression of CD69 on i.v.-transferred violet cells, was detected in the liver that contained only the i.v.-transferred violet cells, but not the Ivag-transferred green cells ( Fig. 3g,h ). Even though the naïve CD8 + T cells were able to be activated in the liver, none of the liver-primed (violet) CD8 + T cells could enter the vaginal mucosa ( Fig. 3f,h ). Direct priming in the vaginal mucosa was further confirmed in a second LN-deficient mouse model, CXCR5 KO mice [40] , in which the Ivag-transferred green cells could be primed locally in vaginal mucosa, while no violet cells from the blood had entered the mucosa ( Supplementary Fig. 3 ). Thus, the data from both WT and LN-deficient mice clearly demonstrated that the Ivag-transferred naïve CD8 + T cells could be primed locally in this type-II mucosa, without any signs of LN immune priming and/or the trafficking of CD8 + T cells through the blood from any other tissue site to the vaginal mucosa. Therefore, we conclude that the naïve CD8 + T cells could be primed locally in the vaginal mucosa independent of LNs, contrary to the well-accepted paradigm. Naïve T-cell vaginal mucosal priming 48 h post Ivag vaccine To characterize the kinetics of immune priming in vaginal mucosa and in draining LNs, we extended our observations to 48 h PI ( Fig. 4a ). In the vaginal mucosa, still containing no violet i.v.-transferred cells, the green Ivag-transferred cells still remained activated, although at a lower level than observed at 24 h PI ( Fig. 4b,d ). In the iliac LN, the violet i.v.-transferred cells started being activated by 48 h, as assessed by the high level of CD69 in the immunized compared with unimmunized mice ( Fig. 4c,d ). The ability to detect priming of violet i.v.-transferred cells in the DLN at 48 h may be due to the migration of vaginal Ag-bearing DCs to the draining LNs by 48 h. Therefore, the Ag-specific immune activation of naive CD8 + T cells could take place in both vaginal mucosa and DLNs at 48 h PI, but also at this time point, priming in the DLN could not account for primed T cells in the vaginal mucosa in the presence of FTY720, as no i.v.-transferred cells were yet able to enter the vaginal mucosa ( Fig. 4b ). Naïve vaginal T-cell priming under physiological conditions The dual-transfer study clearly demonstrated that the immune priming of naïve vaginal CD8 + T cells could be a completely local process ( Figs 3 and 4 ). We further confirmed whether local immune priming could occur in completely intact vaginal mucosa without adoptive transfer of the T cells. We studied the Ag-specific immune activation of vaginal CD8 + T cells in Ivag-immunized Rag-I KO, OT-I transgenic mice ( Fig. 5 ). At 8 h after immunization, the CD69 expression of CD8 + T cells could be detected only in vaginal mucosa but not in DLNs (iliac LNs) ( Fig. 5a,b ) or in any other tissue compartments including axillary LNs, inguinal LNs, spleen and lung ( Supplementary Fig. 4 ). Thus, the CD69-expressing CD8 + T cells detected at 8 h after immunization provided supportive evidence that immune priming is likely to be a local process occurring in the vaginal mucosa but not in the DLNs. In contrast, only at 12 h after immunization, priming was starting to occur in the DLNs ( Fig. 5a,b ). Thus, the kinetics support our conclusion from the dual-transfer studies ( Figs 3 and 4 ) that priming can occur directly in the vaginal mucosa without requiring migration of cells primed in the DLN. Also, we see again that priming in the DLN occurs later than in the mucosa. To further confirm that the CD69-expressing CD8 + T cells originated from the phenotypically naïve cells (CD62L + and CD44 low population) that were the majority (86.5%±2.4%; mean±s.e.m.) of total vaginal CD8 + T cells in unimmunized OT-I mice ( Fig. 5c , left plots and Fig. 5d ), we checked the CD62L and CD44 expression on the CD69-expressing CD8 + T cells in the vaginal mucosa of both naïve and immunized animals ( Fig. 5c right plots and Fig. 5e ). In the immunized animals at 8 h PI, the percentage of naïve cells among total vaginal CD8 + T cells dropped down to 62.1%±1.2% (mean±s.e.m. ), which was significantly lower ( P =0.0009 by a Student’s t -test) than that of unimmunized animals ( Fig. 5c , left plots and Fig. 5d ). More importantly, among the subset that expressed the CD69 activation marker, the percentage of CD44 low and CD62L + cells out of the total CD69-expressing CD8 + T cells was 50.6%±1.4% (mean±s.e.m. ), which was significantly higher ( P =0.0012 by a Student’s t -test) than that of naïve animals (5.3%±5.3%; mean±s.e.m. ; Fig. 5c right plots and Fig. 5e ). Therefore, the CD69 was expressed mostly by the vaginal CD8 + T cells with the naïve phenotype (CD62L + and CD44 low ) that had not yet downregulated CD62L or upregulated CD44 at 8 h after immunization, but not CD8 + T cells with the memory phenotype (CD62L − and CD44 high ). This shows that the primed cells are derived from the naïve population and not the tiny fraction of memory cells in the unimmunized mucosa. Taken together, this experiment confirmed that the local immune priming can occur on the naïve endogenous CD8 + T cells that naturally migrate into the physiologically intact vaginal mucosa before any priming occurs in the DLN. 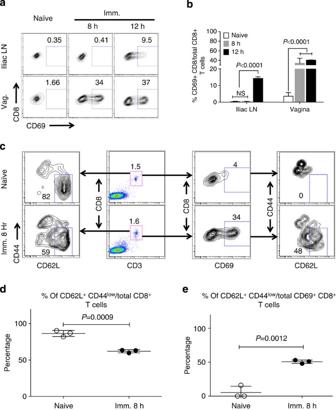Figure 5: The local immune priming of endogenous CD8+T cells that naturally migrate into the physiologically intact vaginal mucosa. The phenotype of endogenous vaginal CD8+T cells in the Ivag SIINFEKL-immunized RAG-I KO, OT-I transgenic mice. This is representative of two independently repeated experiments (n=3) with the same results. (a,b) The CD69 expression of CD8+T cells in vaginal mucosa and iliac LNs of naïve and immunized animals, which were killed at 8 and 12 h PI. (a) Gating strategy. (b) The statistical difference (mean±s.e.m.) among the naïve and the two immunized groups. ThePvalue was generated using a one-way analysis of variance plus Tukey’s multiple comparison. (c) The gating strategies for the phenotype assay of vaginal CD8+T cells in naïve and immunized animals at 8 h after immunization. Left plots, the percentage of CD62L+and CD44lowcells out of total vaginal CD8+T cells. Middle left plots, the percentage of vaginal CD8+T cells. Middle right plots, the percentage of CD69-expressing cells out of total vaginal CD8+T cells. Right plots, the percentage of CD62L+CD44lowcells out of total CD69-expressing vaginal CD8+T cells. (d) The statistical difference (mean±s.e.m.) ofc, left plots. (e) The statistical difference (mean±s.e.m.) ofc, right plots. ThePvalues were generated using Student’st-test. Imm., immunized. Figure 5: The local immune priming of endogenous CD8 + T cells that naturally migrate into the physiologically intact vaginal mucosa. The phenotype of endogenous vaginal CD8 + T cells in the Ivag SIINFEKL-immunized RAG-I KO, OT-I transgenic mice. This is representative of two independently repeated experiments ( n =3) with the same results. ( a , b ) The CD69 expression of CD8 + T cells in vaginal mucosa and iliac LNs of naïve and immunized animals, which were killed at 8 and 12 h PI. ( a ) Gating strategy. ( b ) The statistical difference (mean±s.e.m.) among the naïve and the two immunized groups. The P value was generated using a one-way analysis of variance plus Tukey’s multiple comparison. ( c ) The gating strategies for the phenotype assay of vaginal CD8 + T cells in naïve and immunized animals at 8 h after immunization. Left plots, the percentage of CD62L + and CD44 low cells out of total vaginal CD8 + T cells. Middle left plots, the percentage of vaginal CD8 + T cells. Middle right plots, the percentage of CD69-expressing cells out of total vaginal CD8 + T cells. Right plots, the percentage of CD62L + CD44 low cells out of total CD69-expressing vaginal CD8 + T cells. ( d ) The statistical difference (mean±s.e.m.) of c , left plots. ( e ) The statistical difference (mean±s.e.m.) of c , right plots. The P values were generated using Student’s t -test. Imm., immunized. Full size image DC-dependent activation of naïve T cells in vaginal tissue To completely isolate vaginal mucosa from all the other tissue compartments, we developed a vaginal tissue culture system ( Fig. 6a ). To detect the presence in the vaginal mucosa of APCs that had taken up Ag after Ivag immunization and could prime naïve T cells, we Ivag immunized mice with SIINFEKL peptide and resected the vaginal tissue at day 1 PI ( Fig. 6a ). The vaginal tissue was digested in medium containing collagenase and DNase followed by CD8 depletion to remove any endogenous CD8 + T cells primed either within the vaginal mucosa or in the DLNs followed by vaginal homing ( Fig. 6a ). We co-cultured the CD8-depleted vaginal tissue together with CFSE-labelled naïve OT-I CD8 + T cells for 4 days without adding any Ag to the culture ( Fig. 6a ) and tested Ag-specific CD8 + T-cell proliferation by measuring CFSE dilution of the T cells cultured with the immunized vaginal tissue compared with those cultured with unimmunized vaginal tissue. Being co-cultured with the immunized vaginal tissue, naïve OT-I CD8 + T cells underwent substantial proliferation as compared with those co-cultured with tissue from unimmunized mice ( Fig. 6b,c ). Moreover, if CD11c + cells (including DCs) were depleted from the immunized vaginal tissue, the proliferation of OT-I CD8 + T cells was largely lost ( Fig. 6b,c ). Similarly, the cultures containing both immunized vaginal tissue and naïve OT-I CD8 + T cells showed significantly higher levels of IFN-γ that was also dependent on the presence of CD11c + cells that had taken up Ag during Ivag immunization ( Fig. 6d ). Therefore, the activation of naïve CD8 + T cells in the vaginal tissue required local vaginal APCs that were able to take up Ag at the time of Ivag immunization and then present it later to naïve CD8 + T cells locally in the vaginal mucosa, without the benefit of LNs (not present in these vaginal tissue preparations). 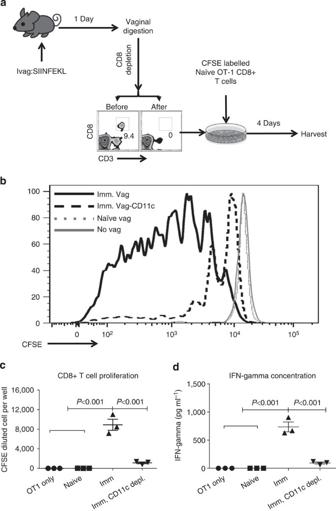Figure 6: The naïve OT-I CD8+T cells activated in surgically resected vaginal tissue. (a) The experimental design. (b) The CFSE dilution of naïve OT-I CD8+T cells in each culture. (c) The absolute number (mean±s.e.m.) of CFSElowcells in each culture. (d) The IFN-γ concentration (mean±s.e.m.) in the supernatant of each culture. This is representative of two independently repeated experiments (n=3 per group of culture containing the pool of three digested vaginal tissues) with the same results.Pvalues were generated using a one-way analysis of variance plus Tukey’s multiple comparison. Imm., immunized. Figure 6: The naïve OT-I CD8 + T cells activated in surgically resected vaginal tissue. ( a ) The experimental design. ( b ) The CFSE dilution of naïve OT-I CD8 + T cells in each culture. ( c ) The absolute number (mean±s.e.m.) of CFSE low cells in each culture. ( d ) The IFN-γ concentration (mean±s.e.m.) in the supernatant of each culture. This is representative of two independently repeated experiments ( n =3 per group of culture containing the pool of three digested vaginal tissues) with the same results. P values were generated using a one-way analysis of variance plus Tukey’s multiple comparison. Imm., immunized. Full size image Local expansion of Ag-specific CD8 T cells in vaginal mucosa We also asked whether the vaginal mucosa could support the local expansion of Ag-specific CD8 + T cells. We characterized the kinetics of CD8 + T-cell immune responses by measuring the tetramer-positive CD8 + T cells at different time points after Ivag immunization with rAd5-gp140 ( Supplementary Fig. 5a ). Day 7 was the earliest time point at which we could detect Ag-specific CD8 + T cells in both the vaginal mucosa and the draining iliac LNs ( Supplementary Fig. 5b ). We therefore decided to block T-cell egress from LNs by FTY720 treatment starting from day 5 PI ( Fig. 7a ). The FTY720 treatment decreased blood Ag-specific CD8 + T cells to a background level, similar to that in either naïve animals or the immunized animals sacrificed at day 5 PI ( Fig. 7b ). In contrast, a similar amount of Ag-specific CD8 + T cells were found in vaginal mucosa of FTY720-treated as untreated immunized mice ( Fig. 7c ). To determine whether the rAd5-gp140 Ivag immunization could induce the formation of IVALT similar to that seen in rAd5-SIINFEKL immunized animals ( Fig. 1d ), we examined vaginal tissue sections of immunized mice either with or without FTY720 treatment by IHC ( Fig. 7d ). The formation of IVALT containing CD3 + , CD8 + and CD11c + cells was observed in the immunized animals either treated or untreated with FTY720. Because the FTY720 treatment diminished the number of Ag-specific CD8 + T cells to a background level in the bloodstream ( Fig. 7b ), which is the only pathway through which the primed T cells can enter the vaginal mucosa from other tissue compartments, we concluded that the quantity of vaginal Ag-specific immune CD8 + T cells as well as the capability of IVALT formation did not depend on blood replenishment. 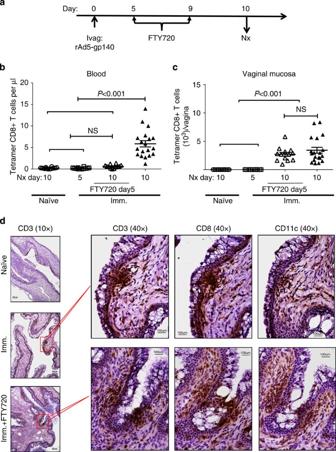Figure 7: Local formation of Ag-specific IVALT in the vaginal mucosa of Ivag-immunized WT mice. (a–c) The absolute number of Ag-specific CD8+T cells in blood and vaginal mucosa of naïve and immunized mice either with or without FTY720 treatment.○, naïve mice euthanized at day 10 PI (n=12); □, immunized mice euthanized at day 5 PI (n=12);▵, FTY720-treated immunized mice euthanized at day 10 PI (n=12);▴, immunized mice euthanized at day 10 PI (n=18). This is the pool of three independently repeated experiments with the same results. (a) The experimental design. (b) The absolute number (mean±s.e.m.) of Ag-specific CD8+T cell in blood. (c) The absolute number (mean±s.e.m.) of Ag-specific CD8+T cell in vaginal mucosa. ThePvalues were generated using one-way analysis of variance plus Tukey’s multiple comparison. (d) Representative IHC staining showing the formation of immune cell clusters containing CD3+, CD8+and CD11c+cells in immunized mice either with or without FTY720 treatment. Scale bar: 100 μm in × 40 photomicrographs; 400 μm in × 10 photomicrographs. Imm., immunized. Figure 7: Local formation of Ag-specific IVALT in the vaginal mucosa of Ivag-immunized WT mice. ( a – c ) The absolute number of Ag-specific CD8 + T cells in blood and vaginal mucosa of naïve and immunized mice either with or without FTY720 treatment. ○ , naïve mice euthanized at day 10 PI ( n =12); □, immunized mice euthanized at day 5 PI ( n =12); ▵ , FTY720-treated immunized mice euthanized at day 10 PI ( n =12); ▴ , immunized mice euthanized at day 10 PI ( n =18). This is the pool of three independently repeated experiments with the same results. ( a ) The experimental design. ( b ) The absolute number (mean±s.e.m.) of Ag-specific CD8 + T cell in blood. ( c ) The absolute number (mean±s.e.m.) of Ag-specific CD8 + T cell in vaginal mucosa. The P values were generated using one-way analysis of variance plus Tukey’s multiple comparison. ( d ) Representative IHC staining showing the formation of immune cell clusters containing CD3 + , CD8 + and CD11c + cells in immunized mice either with or without FTY720 treatment. Scale bar: 100 μm in × 40 photomicrographs; 400 μm in × 10 photomicrographs. Imm., immunized. Full size image To identify the proliferating Ag-specific CD8 + T cells within the vaginal mucosa, we treated the immunized mice from day 5–9 with bromodeoxyuridine (BrdU), a synthetic thymidine analogue that can be incorporated into newly synthesized DNA during cell proliferation ( Fig. 8a ). At day 10 PI, the amount of BrdU + Ag-specific CD8 + T cells in the vaginal mucosa was similar in both FTY720-treated and -untreated immunized groups ( Fig. 8b ), independent of trafficking from LNs. In contrast, the FTY720 treatment caused a significant increase of BrdU + Ag-specific CD8 + T cells in the iliac LNs due to blockage of T-cell egress from DLNs ( Fig. 8b ). Thus, similar to what is found in the lung [41] , the type-II vaginal mucosa can support Ag-specific CD8 + T-cell local expansion that largely contributed to the quantity (the absolute number of Ag-specific CD8 + T cells) and the quality (the formation of IVALT) of vaginal Ag-specific CD8 + T immunity, independent of systemic T-cell recruitment. 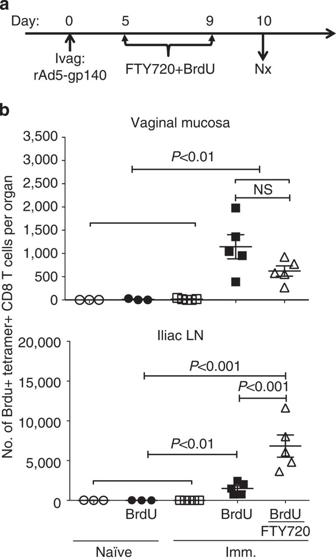Figure 8: The local proliferation of endogenous Ag-specific CD8+T cells in the vaginal mucosa of Ivag-immunized WT mice with or without FTY720 treatment. The BrdU+Ag-specific CD8+T cells in vaginal mucosa of FTY720-treated or -untreated immunized mice.○, naïve mice (n=3); ·, BrdU-treated naïve mice (n=3); □, immunized mice (n=5); ▪, BrdU-treated immunized mice (n=5);▵, FTY720 and BrdU-treated immunized mice (n=5). This is representative of two independently repeated experiments with the same results. (a) The experimental design. (b) The absolute number (mean±s.e.m.) of BrdU+Ag-specific CD8+T cells in vaginal mucosa and iliac LNs. ThePvalues were generated using a one-way analysis of variance plus Tukey’s multiple comparisons. Imm., immunized. Figure 8: The local proliferation of endogenous Ag-specific CD8 + T cells in the vaginal mucosa of Ivag-immunized WT mice with or without FTY720 treatment. The BrdU + Ag-specific CD8 + T cells in vaginal mucosa of FTY720-treated or -untreated immunized mice. ○ , naïve mice ( n =3); ·, BrdU-treated naïve mice ( n =3); □, immunized mice ( n =5); ▪, BrdU-treated immunized mice ( n =5); ▵ , FTY720 and BrdU-treated immunized mice ( n =5). This is representative of two independently repeated experiments with the same results. ( a ) The experimental design. ( b ) The absolute number (mean±s.e.m.) of BrdU + Ag-specific CD8 + T cells in vaginal mucosa and iliac LNs. The P values were generated using a one-way analysis of variance plus Tukey’s multiple comparisons. Imm., immunized. Full size image In the present study, our results demonstrated for the first time that the vaginal mucosa can support the Ag-specific immune priming of naïve T cells and promote Ag-specific T-cell local expansion, despite the absence of MALT or secondary lymphoid tissues. Therefore, in addition to the known role of DLNs, the type-II vaginal mucosa can also act as an inductive site for the generation of primary CD8 + T-cell mucosal immune responses independent of the DLNs, contrary to accepted belief. The priming of immune responses in type-II mucosa is thought to occur only in secondary lymphoid tissues, such as DLNs where the APC-primed naïve T cells can become memory T cells and traffic back to the mucosal sites. However, in direct contrast to this existing widely believed paradigm, we have shown vaginal Ag-specific CD8 + T-cell immune responses are possible following primary Ivag vaccination in mice lacking DLNs ( Fig. 1 ). In agreement with our finding is a recent study by Roth et al . [13] who reported the induction of HSV-specific immune responses in the vagina of LN-deficient LTαKO mice. Further, the priming of CD8 + T cells in the absence of LN involvement has been reported in the lungs (in type I mucosa) [1] , [2] , [3] and other non-lymphoid organs, such as the liver [30] , [31] . Indeed, in our study, we also show the induction of CD8 + T-cell priming in the liver ( Fig. 3g,h ). Moyron-Quiroz et al . [1] , [2] showed that the induction of CD8 + T cells in the lungs without LN involvement may occur in induced bronchial-associated lymphoid tissues in type I mucosa. Likewise, in this study, we demonstrate by IHC the formation of IVALT in the vaginal mucosa following primary IVag vaccination. Similar induction of IVALT has been reported in hormone treated, TK − HSV-vaccinated mice that are challenged with WT HSV [15] . Despite previous studies showing immune protection in the mice without LNs [1] , [2] , [3] , [13] and the presence of IVALT [15] , none of those studies were able to definitively demonstrate the primary immune inductive site because they did not exclude the possibilities that the immune priming can occur in other non-lymphoid organs, such as liver and traffic to the vagina. By using the dual-transfer model to exclude trafficking from these or any other sites through the bloodstream, we have now been able to definitively demonstrate that the vaginal type-II mucosa acts as an inductive site for primary CD8 + T-cell immunity. Therefore, our results demonstrated a new paradigm of IVALT-associated local primary immune induction in type-II mucosa (that lacks structured lymphoid tissues), which is totally independent of any structured lymphoid and/or even non-lymphoid tissues outside vaginal mucosa. These results also demonstrate the ability to induce local vaginal immunity more rapidly than could occur if time were required for DCs to carry Ag to the DLNs and then for T cells to migrate back through the blood to the mucosa. As we have seen in the dual-transfer studies, the latter pathway requires additional time ( Fig. 3e versus Fig. 4d ). This was confirmed in the kinetic study in unmanipulated mice ( Fig. 5a,b ). This kinetic difference has important implications for vaccine delivery strategies aimed at acute protective immunity. Since the number of endogenous naïve T cells specific to any one peptide–major histocompatibility complex complex is extremely small (20–200 per mouse) [42] , it is almost impossible to detect a reliable population of Ag-specific T cells before clonal expansion, after which the Ag-specific T cells are not naïve anymore. To test our hypothesis, we characterized vaginal local immune priming of naïve CD8 + T cells by the Ag-specific activation of CD44-depleted Rag −/− OT-1 CD8 + T cells [43] isolated from the spleen of naïve animals ( Fig. 3a ), because OT-1 or similar TCR transgenic T cells are the only source of naïve CD8 + T cells of a homogeneous Ag specificity. The adoptively transferred OT-1 CD8 + cells have been widely used and accepted as naïve Ag-specific T cells by many experienced labs, in which the investigators published their studies using the transferred cells from unimmunized transgenic mice as naïve [44] , [45] , [46] , [47] , [48] , [49] , [50] , [51] , [52] , [53] , often even without further purification for CD62L high and CD44 low cells. In the current study, we depleted all the CD62L low and CD44 high cells right before the adoptive transfer and brought the purity of our transferred naïve CD8 + T cells up to 98.5% ( Fig. 3a ). Using the dual-transfer model providing a large amount of naïve T cells at the local site, we could detect early immune priming at 24 h PI, which is too short for the primed endogenous naïve T cell to reach a detectable level, most likely through clonal expansion. The rapid detection of response by TCR transgenic T cells due to the greater numbers of Ag-specific cells without an expansion phase is therefore critical to carry out such studies, but does not bear on their naïve status. We, like many other investigators studying vaginal mucosal immunology [12] , [13] , [15] , [21] , [22] , [26] , [54] , treated all the experimental animals with Depo-Provera, a long-acting progesterone, because vaginal Ag-specific CD8 + T-cell immunity could not be consistently induced in animals without Depo-Provera treatment. In contrast to humans, the mouse passes through 4 oestrous stages during an oestrous cycle that lasts only 4 days and then repeats: proestrus, oestrus, metestrus and dioestrus [55] . Among the 4 stages, more CD8 + T cells have been found present in vaginal mucosa during dioestrus [56] . Although the detailed mechanisms of Depo-provera effects on vaginal mucosal immunity remain to be clearly determined, the use of Depo-provera, the dominant hormone in dioestrus, has been shown to affect the thickness of vaginal epithelium [22] , the forming of IVALT [15] , [54] and the accumulation of CD11c + cells [22] . We think the use of Depo-provera, through the regulation of multiple immune parameters, may make the vaginal mucosa more suitable to our Ivag immunization. Without such synchronization of mice that otherwise undergo rapid cyclic changes, it is impossible to carry out controlled studies of vaginal immunity. It is well accepted that T-cell-mediated local protective immunity can play an important role to control the viral infection in peripheral tissue compartments [11] , [24] , [25] , [26] . In addition to the cytotoxic effects based on direct cell-to-cell contact, the tissue-resident T memory cells (T RM ) have been recently found to undergo local development in skin [57] and possess more protective immune functions including the triggering of tissue-wide innate and adaptive immune responses [58] , [59] . Therefore, a goal should be a more efficient vaccine strategy, which can generate strong local T-cell-mediated immune responses [60] without widespread systemic immune activation that facilitates the replication of some viruses, such as HIV and SIV [61] , [62] . Because the DLNs are not required to induce vaginal immunity, it may be possible to induce local immunity without systemic immune activation. Our study outlines definitive evidence for the induction of primary immune induction in vaginal type-II mucosa, thereby identifying a new pathway of vaccine-induced mucosal immunity and a new rationale for the design of future mucosal vaccine strategies. Mice Because this was a study of vaginal immunity, all mice used in the current study were females from 16–20 weeks of age. BALB/c and C57BL/6 mice were purchased from NCI animal facility (Frederick, MD). OT-1, LTα KO and CXCR5 KO mice (all with C57BL/6 background) were purchased from Jackson Laboratories (Bar Harbor, ME). All experimental protocols were approved by and carried out under the guidelines of the NCI’s Animal Care and Use Committee. All the animals were grouped randomly and the number of animals in each group is equal to or greater than 3 ( n ≥3). All the experiments were repeated at least two (two to four) times. Reagents and inocula Replication-deficient adenovirus 5-expressing HIVgp140 (rAd5-gp140) was developed and kindly provided by Dr Gary Nabel (Vaccine Research Center, NIAID, Bethesda MD). Replication-deficient adenovirus 5-expressing SIINFEKL (rAd5-SIINFEKL) was first developed by Dr S.E. Hensley in Jon Yewdell’s and Jack Bennink’s laboratory (NIAID) and kindly provided by Dr Robert Seder in (NIAID). The FTY720 was purchased from Cayman Chemical (Ann Arbor, MI). The SIINFEKL peptide was purchased from Polypeptide Laboratory (San Diego, CA). The mutant E. coli labile toxin (mLT) was a kind gift of Dr John Clements (Tulane University, New Orleans). The DOTAP and BrdU were purchased from Sigma (St Louis, MO). The Depo-provera was purchased from the Department of Veterinary Medicine, NIH. Intravascular T-cell staining Alexa fluor-647 labelled anti-mouse Thy1.2 antibody was diluted in PBS at 250 ng ml −1 . Each mouse was injected with 100 μl of diluted antibody through the tail vein. All the animals were euthanized at 1 min post i.v. injection, a time point at which all the blood T cells in retro-orbital sinus were Thy1.2 positive. Dual transfer The CD8 + T cells were isolated from Rag −/− OT-1 TCR transgenic mice using a CD8 isolation kit (Miltenyi Biotec, Auburn, CA). The CD44 + cells were depleted using biotinylated anti-mouse CD44 (1:2,000 dilution, BioLegend, San Diego, CA) and anti-biotin beads (Miltenyi Biotec). The naïve CD8 + OT-1 T cells were labelled with either CFSE or violet dye (both from Invitrogen, Grand Island, NY) at 5 μM. Ten microlitres of CFSE-labelled cells (1 × 10 8 ml −1 ) were directly injected into the vaginal tissue (Ivag) using a Hamilton syringe with a 32G needle. One hundred microlitres of violet dye-labelled cells (1 × 10 7 ml −1 ) was injected into the tail vein (i.v.). The mice were under isoflurane general anaesthesia during the performance of dual transfer. Immunization All the immunizations in this study were performed Ivag. The dose of each inoculum was: 2 × 10 7 p.f.u. of rAd5-gp140, 1 × 10 7 of rAd5-SIINFEKL or 40 μg of SIINFEKL peptide plus 5 μg of mutant E. coli labile toxin (mLT) and equal volume of DOTAP. Ivag immunizations were performed using a 20-μl pipette tip to apply the inoculum into the vaginal canal atraumatically. All the immunized mice were maintained under inhalation anaesthesia for 20 min. Vaginal tissue culture The resected vaginal tissue was digested in RPMI 1640 medium (GIBCO, Grand Island, NY) containing collagenase-D (400 U ml −1 , Roche Indianapolis, IN), DNase-I (2.5 mg ml −1 , Roch), Penicillin–Streptomycin (100 μg ml −1 , GIBCO), HEPES buffer (20 mM, GIBCO) and fetal bovine serum (10%, GIBCO). The digestion lasted for 20 min with stirring. The vaginal tissue was then smashed through a 70-μm cell strainer (Fisher, Pittsburgh, PA) followed by CD8 depletion using Dynal Beads (Life Technologies). The CD8-depleted vaginal tissue, either with or without CD11c-depletion (CD11c kit, Miltenyi Biotec), was co-cultured with 1 × 10 6 CFSE (Invitrogen)-labelled naïve OT-1 CD8 + T cells in RPMI medium containing Penicillin–Streptomycin (100 μg ml −1 , GIBCO), HEPES buffer (10 mM, GIBCO), L -glutamine (2 mM, GIBCO), gentamicin (50 mg ml −1 , Sigma), MEM non-essential amino acid (GIBCO), sodium pyruvate (1 mM, GIBCO), 2-mercaptoethanol (10 μM, Sigma), fungizone (2.5 μg ml −1 , GIBCO) and fetal bovine serum (20%, GIBCO). Antibodies and flow cytometry Anti-mouse CD3, CD8, CD69, CD44, CD25 and CD62L were purchased from Biolegend and used to stain the cells at the concentration of 150 ng ml −1 . Data were collected using a LSRII using DIVA software (BD Biosciences, San Jose, CA) or a FACSCalibur flow cytometer using CellQuest software (BD Biosciences). The analysis of data was performed using FlowJo (Tree Star, Ashland, OR). Depo-Provera synchronization All the mice in our study received Depo-Provera at a dose of 3 mg per mouse through subcutaneous injection 5 days before each experiment. FTY720 treatments FTY720 was given by IP injection at an initial dose of 50 μg per mouse followed by daily maintenance injection at a dose of 5 μg per mouse. Bromodeoxyuridine (BrdU) treatment and staining The BrdU (1 mg per mouse, Sigma) was given by daily intraperitoneal injections for 5 days. The staining of BrdU-positive cells was performed using a Brdu staining kit (BD Biosciences) according to the manufacturer’s instructions. Immunohistochemistry The vagina was embedded in optimal cutting temperature compound (O.C.T.) and snap frozen in liquid nitrogen precooled isopentane. Frozen vaginal tissue blocks were cut into sections with a thickness of 5 μm, stored in −70 °C until use. Cryostat sections were fixed in acetone for 5 min, rehydrated in PBS and incubated overnight with primary antibodies including rabbit anti-mouse CD3 (1:100 dilution, AbCam), rat anti-mouse CD8 (1:200 dilution, Biolegend) and hamster anti-mouse CD11c (1:150 dilution, Biolegend). The primary antibodies were washed out three times by PBS followed by the addition of HRP-conjugated secondary antibodies (Vector Lab) including horse anti-rabbit IgG, goat anti-rat IgG and goat anti-hamster IgG. The secondary antibodies were incubated in room temperature for 30 min followed by DAB (kit from Vector Lab) development and hematoxylin (BBC Biochemical) counter staining. Statistics The statistics of this study was performed using Prism software. One-way analysis of variance plus Tukey’s multiple comparison was used to compare multiple groups; Student’s t -test was used to compare two groups. How to cite this article: Wang, Y. et al . Vaginal type-II mucosa is an inductive site for primary CD8 + T-cell mucosal immunity. Nat. Commun. 6:6100 doi: 10.1038/ncomms7100 (2015).